Methane hydrate formation in confined nanospace can surpass nature Natural methane hydrates are believed to be the largest source of hydrocarbons on Earth. These structures are formed in specific locations such as deep-sea sediments and the permafrost based on demanding conditions of high pressure and low temperature. Here we report that, by taking advantage of the confinement effects on nanopore space, synthetic methane hydrates grow under mild conditions (3.5 MPa and 2 °C), with faster kinetics (within minutes) than nature, fully reversibly and with a nominal stoichiometry that mimics nature. The formation of the hydrate structures in nanospace and their similarity to natural hydrates is confirmed using inelastic neutron scattering experiments and synchrotron X-ray powder diffraction. These findings may be a step towards the application of a smart synthesis of methane hydrates in energy-demanding applications (for example, transportation). Natural methane hydrates are crystalline solids that form when methane and water comes into contact under thermodynamically favourable conditions, that is, high pressure (typically more than 6 MPa) and relatively low temperature (slightly below room temperature), giving rise to an ice-like hydrogen-bonded structure [1] . Under these conditions, natural hydrates crystallize in a cubic structure known as type sI. This structure is constituted by cages of two different types: (i) six large cages having 12 pentagonal and 2 hexagonal faces (denoted by 5 12 6 2 ) formed by 24 water molecules and (ii) two small cages having 12 pentagonal faces (denoted by 5 12 ) formed by 20 water molecules [2] . These cages have an average cavity radius of 0.433 and 0.395 nm, respectively, which is enough to host one methane molecule per cage, resulting in a nominal stoichiometry 1CH 4 ·5.75 H 2 O. Actual prospections have estimated vast deposits of methane hydrates in deep-sea sediments and the permafrost (that is, the estimated amount of methane contained in the form of hydrates in the southern US Atlantic margin is as high as 30 billion metric tons (Gt) [3] , [4] . Actual depletion of fossil fuel reserves all around the world has addressed the attention of governments and scientists towards natural methane hydrates reservoirs, based on the assumption that they could be a major energy resource in the near future (if 100% of the cavities are filled with methane, one volume of hydrate would dissociate into a maximum of 180 volumes (STP) of methane). The amount of energy in the form of hydrate may be twice that of all other fossil fuels combined [4] . Methane, the major component of natural gas (NG), has high hydrogen to carbon ratio and it involves both a greater energy density per unit mass and less carbon dioxide emissions (around 40% less) during combustion than gasoline or diesel. These properties led to the nomination of NG as premium fuel in a low-carbon energy future. Actual technology for NG storage is based either on compressed natural gas (CNG), in automobile industry, or on liquefied natural gas (LNG), for large distance transportation. Despite the large energy density of these technologies, mainly liquefied NG, the use of high pressure (25 MPa and 25 °C) or low temperature (−162 °C and 0.1 MPa) becomes undesirable from the safety and energy saving view. An alternative solution concerns the use of porous materials to store NG (adsorbed natural gas (ANG)) at a similar high density, but substantially lower pressure. Unfortunately, actual storage on porous solids, mainly metal-organic frameworks and carbon materials, exhibits certain limitations, at least in a gravimetric basis, to fulfil the new methane program from the US Department of Energy (see DOE MOVE program at https://arpa-e-foa.energy.gov ) [5] , [6] , [7] , [8] , [9] , [10] . As described above, methane hydrates are constituted by methane molecules entrapped (typically one molecule per cavity) within hydrogen-bonded water cavities. When a small molecule like methane is encaged in hydrates, the guest methane molecules are separated ca . 0.5 nm by the water cages, that is, the energy density in hydrates is approximately the same as that of the compressed gas (that is, methane gas at 0 °C and 18 MPa). Taking into account these premises, NG storage and transportation in the form of gas hydrates could be envisaged as a promising alternative, provided that they can be synthesized under mild conditions (low pressures and mild temperatures) and within reasonable time scale. With this in mind, here we report the nucleation and growth of methane hydrates in the confined nanospace of activated carbons. High-pressure methane adsorption measurements show that these nanostructures can be synthesized under mild conditions, with ultrafast kinetics and with a stoichiometry that mimics nature. The formation of methane hydrate nanocrystals with sI structure is confirmed for the first time by using inelastic neutron scattering (INS) experiments and synchrotron X-ray powder diffraction (XRPD). These results provide some bright light into the formation mechanism and into the prospective of this promising field. Methane hydrate formation in activated carbon Methane adsorption experiments either in wet or dry conditions were carried out using a petroleum pitch-derived activated carbon, labelled PP-AC. It is worth mentioning some of the characteristics of this sample to better understand the adsorption behaviour [11] . The pore walls of the PP-AC consist of wrinkled graphenes that infers efficient slit-shaped pores, as it can be observed in Supplementary Fig. 1 . The well-developed graphene layers being quite different from conventional activated carbon can be clearly observed [12] , [13] . The PP-AC sample exhibits a large surface area, around 3,670 m 2 g −1 , and a total pore volume ( V t ) of 2.44 cm 3 g −1 . Micropore ( V 0 ) and mesopore ( V meso ) volume in the PP-AC sample deduced from the nitrogen adsorption isotherm at −196 °C are 1.20 and 1.24 cm 3 g −1 , respectively. Pore size distribution after application of the quenched solid density functional theory method to the nitrogen adsorption data reflects that sample PP-AC contains a well-defined micro- (25%) and mesoporous (75%) structure with a narrow peak at 1 nm and a wide shoulder with peak maxima at 2 and 3 nm (see Supplementary Fig. 1 ). In addition, mercury porosimetry shows a wide macropore size distribution, ranging 0.1–100 μm, with a maximum at 10 μm. The presence of highly developed porous structure combining micro-, meso- and macropores would be of paramount importance to elucidate the hydrate formation mechanism on confined nanospaces. Water adsorption isotherm of PP-AC at 25 °C is reported in Supplementary Fig. 2 . At low relative pressures, the amount adsorbed is nil, as corresponds to a hydrophobic material. Condensation takes place at high relative pressures ( p / p 0 >0.8) with a saturation capacity of 1.8 g g −1 of dry carbon, corresponding to a 93% filling of the total pore volume (under the assumption that density of the adsorbed water is 1.0 g cm −3 ). The water adsorption isotherm has a remarkable hysteresis loop that comes from a metastable assembly structure of water in the adsorption branch [14] , [15] . Our initial hypothesis would be that the small thickness of the metastable water layer (that provides a very high-interfacial liquid water–methane contact area), together with the low interaction of water molecules with the hydrophobic carbon surface could speed up the methane hydrate formation process [16] , [17] . Consequently, the methane hydrate formation on sample PP-AC was examined for different amounts of adsorbed water. The available nanoporosity of water-adsorbed PP-AC sample was measured by N 2 adsorption at −196 °C after freezing water adsorbed in nanopores ( Supplementary Fig. 3 ). Here we introduce the weight ratio of adsorbed water to carbon, R w ; R w =1.8 corresponds to fully saturated pores with water. The R w was changed up to R w =4.1, that is, from unsaturated samples ( R w of 0.6 and 1.1) to oversaturated samples ( R w of 2.9 and 4.1). Supplementary Figure 3 shows that the larger the R w the lower the residual porosity is. For R w of 0.6 and 1.1, the pores are partially filled with water to 66 and 80% total pore filling (total pore volume measured by nitrogen at −196 °C), whereas for R w superior to 1.8, the pores (micropores and mesopores; see Supplementary Fig. 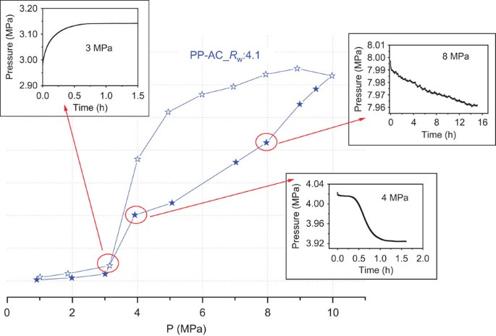Figure 3: Methane hydrates formation kinetics. Pressure change profile for methane until equilibrium at two different points of the adsorption isotherm (4 and 8 MPa) and at one point of the desorption branch (3 MPa) for sample PP-ACRw=4.1 at 2 °C (closed symbols represent adsorption and open symbols represent desorption). 1b ) are almost saturated with water (even macropores must be filled with a metastable water film), in agreement with the water adsorption isotherm. 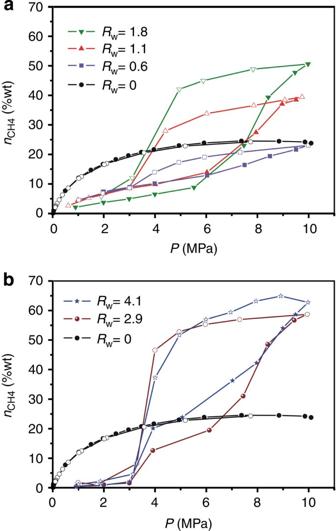Methane adsorption capacity under the water-supplying conditions by varying R w was evaluated using a volumetric apparatus as described in the experimental section. Figure 1: Methane adsorption in the presence of water. Methane adsorption/desorption isotherms at 2 °C for sample PP-AC dry and wet (a)Rw=0.6, 1.1, 1.8; and (b)Rw=2.9, 4.1, in a gravimetric basis (gCH4gdry carbon−1× 100). Closed symbols represent adsorption branch and open symbols represent desorption branch. Figure 1a shows the adsorption isotherms of PP-AC in a gravimetric basis (wt.% methane per weight of dry carbon) for R w 0.6, 1.1 and 1.8 (dry sample was included for the sake of comparison). At this point, it is interesting to highlight that the methane adsorption capacity for the dry carbon at 10 MPa (24 wt.% or 0.24 g g −1 ) is completely reversible and it is among the highest values ever reported in the literature, even if compared with carbons of similar textural properties or metal-organic frameworks [6] , [7] , [8] , [9] , [10] , [18] . Concerning the wet samples and independently of R w , the methane adsorption capacity is low compared with the dry sample at least at low pressures (below 3 MPa), most probably due to pore blocking by preadsorbed water. However, for pressures higher than 3 MPa, the scenario changes completely. In all cases a sigmoidal behaviour can be clearly appreciated, the higher the R w value, the more remarkable the adsorption increment is. All adsorption isotherms exhibit a large hysteresis loop that increases with R w , thus indicating a different adsorption and desorption mechanisms for methane in these samples. In any case, methane is almost completely released below 4 MPa. Figure 1: Methane adsorption in the presence of water. Methane adsorption/desorption isotherms at 2 °C for sample PP-AC dry and wet ( a ) R w =0.6, 1.1, 1.8; and ( b ) R w =2.9, 4.1, in a gravimetric basis (g CH4 g dry carbon −1 × 100). Closed symbols represent adsorption branch and open symbols represent desorption branch. Full size image A closer look to the effect of the coexistent water amount in the adsorption behaviour reflects the presence of a critical R w value above which the adsorption capacity of the wet samples surpasses that for the dry sample, thus suggesting an enhancement role of preadsorbed water in methane adsorption. Previous studies reported in the literature have anticipated the beneficial effect of water on methane adsorption, although a deep evaluation of the adsorption process (adsorption kinetics at different steps, phase identification, chemical stoichiometry and so on) and the adsorption mechanism responsible for this behaviour has not been clearly elucidated [19] , [20] , [21] . Figure 1b shows the methane adsorption isotherms for heavily water-supplied samples with higher R w =2.9 and 4.1 (oversaturated samples). Interestingly, on these samples, in addition to the inflexion point at high pressures (above 6–8 MPa) observed in Fig. 1a , there is an additional adsorption step at relatively lower pressures (around 3 MPa). Despite the scarce number of studies dealing with methane adsorption on wet-activated carbons, to our knowledge, this is the first time that a two-step adsorption process can be discerned for activated carbons. Previous studies described in the literature have only described the sigmoidal shape at 4–6 MPa [19] , [20] , [21] . In addition to the two-step adsorption process, both samples exhibit a large hysteresis loop, the desorption branch being quite stable down to ca. 4 MPa, indicating the formation of the stable phase of the methane and water mixture. The transition of a metastable island state to the stable solid-like state on the adsorption branch with the methane pressure should occur. In fact, the pressure associated with the first jump in the adsorption isotherm perfectly fits with the formation pressure for natural hydrates in bulk water at 2 °C ( P w =3.14 MPa) [1] . Last but not the least, it is important to highlight that the saturated adsorption capacity in both heavily water-supplied samples is extraordinarily large, 59 wt.% (0.59 g g −1 ) and 63 wt.% (0.63 g g −1 ) for R w 2.9 and 4.1, respectively, these values being over twofold the methane adsorption capacity of the dry sample. As described above, these values (on wet and dry samples) constitute the best adsorption capacity values for methane ever reported in the literature [8] , [9] , [10] . Despite the beneficial effect of preadsorbed water on methane adsorption, Supplementary Fig. 4 clearly reflects that the adsorption capacity achieves a plateau with R w , that is, above a certain amount of water supplied, the system does not experience any improvement at all since it behaves like a bulk system. At this point, it is noteworthy to mention that the methane adsorption isotherm on bulk water (in the absence of confinement effects) gives nil adsorption over the whole-pressure range evaluated due to the following: (i) the small gas–liquid interphase and (ii) the slow kinetics of the nucleation and growth of synthetic hydrates, at least in the absence of confined effect as it will be discussed later. Another important factor in the nucleation and growth of synthetic hydrates is the formation temperature. As described above, natural hydrates are formed in nature on demanding conditions of high pressure and low temperature. To evaluate the effect of temperature in the adsorption behaviour reported for water preadsorbed in confined nanopores, sample PP-AC saturated under R w =1.8 was exposed to methane up to 10 MPa at different adsorption temperatures. As it can be observed in Fig. 2 , the amount adsorbed decreases and the hysteresis loop becomes progressively less marked on a slight increase in the adsorption temperature up to 10 °C, where the hysteresis loop completely vanishes. 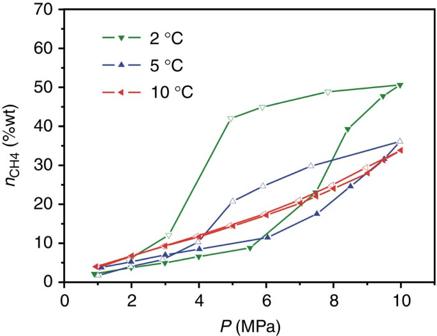This observation suggests that the complex methane adsorption process on confined nanospaces, that is, nucleation and growth of methane hydrates, is highly sensitive to the adsorption temperature, ~2 °C being the upper limit for nucleation. Figure 2: Effect of temperature on methane hydrates formation. Methane adsorption/desorption isotherms for sample PP-AC withRw=1.8 at different adsorption temperatures. Closed symbols represent adsorption branch and open symbols represent desorption branch. Figure 2: Effect of temperature on methane hydrates formation. Methane adsorption/desorption isotherms for sample PP-AC with R w =1.8 at different adsorption temperatures. Closed symbols represent adsorption branch and open symbols represent desorption branch. Full size image The major problem associated with storing methane in the form of hydrates, that is, synthetic methane hydrates, concerns its extremely slow growth kinetics. Indeed, the blank experiment in the absence of confinement effects, that is, in the absence of activated carbon, gives no methane adsorption over the whole-pressure range evaluated (up to 10 MPa). Only under special conditions, for example, water-in-crude oil emulsion, methane hydrate can be formed under realistic time scale (within hours) due to the increase gas–liquid contact area, although using extremely high pressures (10 MPa) [15] , [16] , [22] . Interestingly, these kinetic limitations can be overcome by taking advantage of the confinement effects on carbon nanospaces [23] . It is well known that confinement of materials in nanometre-scale spaces induces unique phenomena in respect to the bulk phase due to the enhanced interaction potential of molecules and ions within the nanospace walls. These phenomena called quasi-high-pressure effect has been used by some of the authors to induce high-pressure gas-phase reactions, that is, production of metallic sulphur one-dimensional chain and KI nanocrystals, at ambient pressure [23] , [24] . To evaluate the effect of the confinement in the hydrate formation kinetics at the two steps of the adsorption process described above, Fig. 3 reports the pressure–time change profile until equilibrium for three different points of the methane adsorption/desorption isotherm on sample PP-AC with R w =4.1, two points corresponding to the adsorption branch (4 and 8 MPa) and one point corresponding to the desorption branch (3 MPa). Figure 3: Methane hydrates formation kinetics. Pressure change profile for methane until equilibrium at two different points of the adsorption isotherm (4 and 8 MPa) and at one point of the desorption branch (3 MPa) for sample PP-AC R w =4.1 at 2 °C (closed symbols represent adsorption and open symbols represent desorption). Full size image Interestingly, the first adsorption step at relatively ‘low pressures’ (4 MPa) is surprisingly fast, pressure reaching equilibrium in <1 h. This observation suggests that the complex adsorption process taking place in this pressure range (possible hydrate formation in large pores) is relatively fast. Longer equilibrium times (around 14 h) are required for the high-pressure points of the isotherms, thus suggesting the presence of certain kinetic restrictions at the methane adsorption stage. Most probably, the first jump in the adsorption isotherm, mainly observed in oversaturated samples, must correspond to methane hydrate formation in large pores (macropores and large mesopores where a metastable water layer is present), this process being relatively fast. Once these structures are formed, excess methane must diffuse throughout the pore network filled by hydrate crystallites to reach the inner pores (small mesopores and micropores), where hydrate nucleation and growth is slightly hindered, thus explaining the different growing kinetics. In summary, these observations suggest that confinement effects on carbon nanopores not only enhance the methane adsorption capacity but rather infer an intensive improvement in the hydration formation kinetics. In situ Ineslatic Neutron Scattering As described along the manuscript, previous studies have anticipated the beneficial effect of water in the methane adsorption capacity of activated carbons [19] , [20] , [21] . Although it has been speculated no evidence of methane hydrate formation has been described in the literature up to date. To dissipate any doubt about the possibility of methane hydrate formation in nanoconfined spaces, in situ INS measurements have been performed at the Rutherford Appleton facilities at the United Kingdom. There is an intrinsic advantage in using INS with hydrogenous materials due to the incoherent scattering cross-section of the proton, which is almost two orders of magnitude greater than in any other nucleus, thus allowing for a relatively simple access to the self-dynamics of molecular hydrogen. INS experiments were performed using D 2 O in spite of H 2 O to reduce parasitic scattering from the water framework. Before any adsorption experiment, a background spectrum was collected to subtract any hydrogen interference from the carbon surface. After the background, deuterated sample was contacted with methane (CH 4 ) at two different pressures (4 and 6 MPa) for 1 h at 2 °C. Shortly after that, the reactor was properly cooled down to −268 °C for the neutron scattering measurements using the TOSCA spectrometer at the Rutherford Appleton facilities. The methane spectrum on dry carbon was also measured for the sake of comparison. 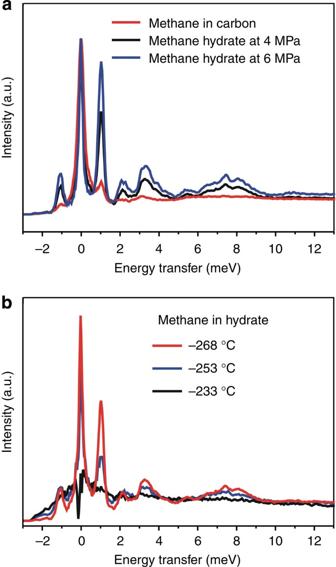Figure 4: Inelastic neutron scattering of methane hydrates. Rotational spectra of hydrogen coming from the methane molecule in wet (deuterated)-activated carbon PP-AC (a) at different pressures and (b) at different temperatures. The spectrum of dry-activated carbon containing 6 MPa methane is included for the sake of comparison. Figure 4a shows the quantum rotational spectra for activated carbon PP-AC dry and wet (deuterated) at 4 and 6 MPa (in the dry sample only 6 MPa was evaluated). As it can be observed in Fig. 4a , methane adsorbed on the dry-activated carbon gives rise only to the elastic peak at an energy transfer of 0 meV. The spectrum of methane in the dry-activated carbon is dominated by its molecular recoil and all spectroscopic information is washed out. This is due to the light mass of methane and the presence of weak intermolecular interactions. However, the situation changes drastically in the deuterated (wet) samples. In this case, the rotational spectra show, in addition to the elastic band described above, additional contributions on both sites due to inelastic scattering of neutrons. When encaged in deuterated ice network, methane molecules behave almost like free rotors even at −268 °C. These inelastic rotational lines appear at energy transfers of E =± 0.99 meV (7.98 cm −1 ), E 1 =2.3 meV (18.54 cm −1 ) and E 2 =3.3 meV (26.61 cm −1 ), independently of the methane pressure applied. The rotational constant of methane as a free rotor is B CH4 = h /2 θ =0.655 meV. The first peak corresponding to the transition from the rotational ground state ( J =0) to the first excitation state ( J =1) should appear at 1.31 meV (10.56 cm −1 ). The shift observed in this peak in our experiment (by 20%) is in accordance with the observations by Tse et al . [25] for synthetic hydrates on non-confined spaces. Other two peaks are assigned to the rotational transitions J =1→ J =2 and J =0→2, respectively. Interestingly, these values are coincident with those found in natural methane hydrates from the Pacific see-floor, in which the methane molecule was considered like an almost free rotor [26] . The almost free rotation of methane is a clear indication that guest molecules occupy positions in the centre of the cages of the hydrate lattice. At off-centre positions, the effect of a non-spherical symmetry potential due to the dipole–octopole interactions would be observed. These peaks above 5 meV are attributed to translational motion of the methane molecule in the two kind of water cages, the small ones denoted as 5 12 and the large ones denoted 5 12 6 2 (ref. 25 ). Consequently, the observation of these inelastic quantum rotational bands is the first direct evidence of methane hydrate formation in the confinement space of nanoporous carbons, even at 4 MPa. The relatively ‘low’ pressure and the relatively fast adsorption kinetics (<1 h) constitute a step stone towards the application of synthetic methane hydrates for methane storage in on-board applications or for overseas transportation. Figure 4: Inelastic neutron scattering of methane hydrates. Rotational spectra of hydrogen coming from the methane molecule in wet (deuterated)-activated carbon PP-AC ( a ) at different pressures and ( b ) at different temperatures. The spectrum of dry-activated carbon containing 6 MPa methane is included for the sake of comparison. Full size image Figure 4b shows the effect of the temperature for the INS measurement on the relative intensity of the rotational transitions. An increase in temperature from −268 to −233 °C gives rise to a line broadening, suggesting the transformation from quantum rotations to translation-coupled rotation, that is, classical rotational diffusion. In situ synchrotron X-ray diffraction To further confirm the methane hydrate formation and to give some insight into the crystal structure of the synthesized nanocrystals, synchrotron XRPD experiments were performed. The XRPD patterns were collected in the high-pressure end station of the MSPD beamline at synchrotron ALBA in Spain using the PP-AC sample oversaturated with D 2 O ( R w =4.1). The spectra of the ‘wet’ sample in the absence of methane and at room temperature exhibit the expected pattern for an amorphous carbon with no well-defined peaks over the whole range evaluated (see Fig. 5a ). Incorporation of 3 MPa of methane at 2 °C, just below the threshold pressure for hydrate formation, gives rise to the characteristic peaks of the hexagonal structure of deuterated ice (denoted by I in the spectra), these peaks being more prominent after a subsequent cooling down to −3 °C. Interestingly, no diffraction peaks attributed to methane hydrate formation were observed under these conditions, in close agreement with the methane adsorption isotherms. The crystallite size of the ice formed was calculated from the peak width after application of the Scherrer equation using a Si standard (NIST material 640c) as a reference. The estimated average crystallite size was 15 nm in both cases, independently of the temperature and the time. 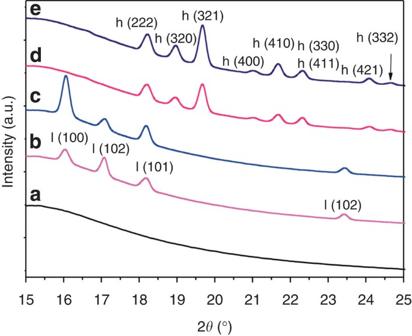Figure 5: X-ray powder diffraction of methane hydrates. Synchrotron XRPD patterns of (a) wet-deuterated activated carbon PP-AC at 25 °C (in the absence of methane), (b,c) wet-deuterated carbon at 3 MPa of methane and 2 and −3 °C, respectively, and (d,e) wet-deuterated carbon at 5 MPa of methane and 2 and −3 °C, respectively. Reflections corresponding to ice and hydrate are market as I and h, respectively, followed by their Miller indices. Figure 5: X-ray powder diffraction of methane hydrates. Synchrotron XRPD patterns of ( a ) wet-deuterated activated carbon PP-AC at 25 °C (in the absence of methane), ( b , c ) wet-deuterated carbon at 3 MPa of methane and 2 and −3 °C, respectively, and ( d , e ) wet-deuterated carbon at 5 MPa of methane and 2 and −3 °C, respectively. Reflections corresponding to ice and hydrate are market as I and h, respectively, followed by their Miller indices. Full size image Subsequently, the sample was heated up to 5 °C until complete melting of the ice (no peaks in the spectra could be observed), and then the capillary was pressurized with methane up to 5 MPa (well above the first pressure threshold) and the temperature was lowered to 2 °C. Under these conditions, new XRPD peaks suddenly appeared (in <10 min), corresponding to the sI structure of the methane hydrate [27] , [28] , [29] . The formation process was completed in 30 min, and peak intensities did not change when continuing the process for another 30 min. Interestingly, a subsequent decrease in the capillary temperature down to −3 °C did not produce any change in the resulting pattern, and no additional ice formation could be observed. This observation suggests that most of the water incorporated into the carbon was involved in the methane hydrate phase. The analysis of the peak widths shows an average crystallite size of 16 nm at both temperatures, very close to the ice crystallite size previously formed. In summary, XRPD measurements constitute the first experimental evidence that methane hydrate sI nanocrystals can be grown in the cavities of activated carbons within minutes by taking advantage of the nanoconfinement effects. The nanocrystals observed under these conditions must correspond to methane hydrates grown in the metastable water layer present on large pores (macropores) with an average crystallite size of 16 nm, which correspond to several unit cells (unit cell of the sI methane structure is 1.2 nm). Gas pressures above 5–6 MPa favours the methane hydrate nucleation and growth in inner cavities (mesopores and wide micropores), with slower kinetics and a marked hysteresis loop, as described above, although these additional nanostructures may not be detected by X-ray measurements due to their limited crystal size in small cavities. Stoichiometry of confined methane hydrates Last but not least, the stoichiometry of the methane hydrates synthesized in the confined nanospace has been estimated from the amount of methane adsorbed at 10 MPa for each R w , taking into account the amount of water adsorbed under each condition. In the case of oversaturated conditions, it is assumed that 1.8 g of water per gram of sample are adsorbed in micro- and mesopores (according to the water vapour adsorption isotherm; see Supplementary Fig. 2 ), whereas the remaining water is placed in larger pores (macropores). In addition, in the oversaturated samples the amount of methane adsorbed has also been split into the two steps of the adsorption isotherm, so that the stoichiometry of the nanostructures can be estimated in the low and in the high-pressure regime. As it can be observed in Table 1 , samples under less saturated conditions exhibit an empirical formula of 1CH 4 ·(3.6–4.1)H 2 O. Taking into account that natural hydrates have a stoichiometry of 1CH 4 ·5.75H 2 O, the under-stoichiometric behaviour at these conditions suggests (i) either the formation of non-stoichiometric hydrates in small pores, due to steric hindrance [30] or (ii) the presence of additional free-adsorbed methane in narrow cavities (below 1 nm), non-forming hydrates. Interestingly, the scenario changes completely for oversaturated samples. In these samples, the empirical formula has been estimated for the two steps in the adsorption isotherm (3–4 MPa range and 6–8 MPa range), that is, the amount of methane adsorbed in each step has been considered independently for the calculations as described above. As observed in Table 1 , the stoichiometry of the structure formed in the first jump is extremely close to natural hydrates 1CH 4 ·(5.3–5.8)H 2 O, corresponding to those hydrates formed in large pores. Concerning the second step in the methane adsorption isotherm (6–8 MPa), a similar under-stoichiometric behaviour is observed, 1CH 4 ·(4.1–4.2)H 2 O. Taking into account the slow kinetics for this process together with the non-stoichiometric behaviour, this observation provides more insight into the adsorption mechanism: methane hydrates in large macropores are formed within minutes above 3 MPa, in close agreement with the stoichiometry and formation pressure of natural hydrates, whereas larger pressures (above 6 MPa) and slower sorption kinetics, within hours, identify the methane hydrate nucleation and growth in smaller pores (mainly mesopores and wide micropores). In any case, the presence of free-adsorbed methane in narrow pores cannot be excluded to explain the non-stoichiometric behaviour. Table 1 Methane hydrate stoichiometry. Full size table We have experimentally identified for the first time the growth of synthetic methane hydrates in the nanospace of carbon materials by using in situ INS measurements and synchrotron XRPD. Quantum rotational spectra (elastic and ineslastic scattering of neutrons) perfectly fit those found in natural methane hydrates from the Pacific see-floor, while XRPD measurements clearly identify the sI structure of methane hydrate. Taking advantage of the confinement effect on carbon nanospaces synthetic hydrates can be prepared under less demanding conditions, thus surpassing nature. Confinement effects allow faster growth kinetics (only a few minutes are required to growth these structures) and lower nucleation pressures (below 4 MPa), while keeping the stoichiometry of natural hydrates (1CH 4 ·5.75 H 2 O). In addition, synthetic hydrates are fully reversible over the whole-pressure range evaluated, with a large working capacity in a ‘narrow’ pressure window, that is, 3–10 MPa. The total methane adsorption capacity in these oversaturated systems is extraordinarily large with value around 59 wt.% (0.59 g g −1 ) and 63 wt.% (0.63 g g −1 ) for samples with R w =2.9 and 4.1, respectively, these values being over twofold the methane adsorption capacity of the dry sample. The large adsorption capacity for methane, the fast kinetics, the complete reversibility of the nucleation and growth process and the large working capacity of these systems under a ‘narrow’ pressure window make methane hydrates grown in confined nanospaces a promising alternative for NG storage and transportation. Sample preparation The nanoporous carbon sample used in the present study was developed using a mesophase pitch prepared by the pyrolysis of a vacuum residue (VR). The pyrolysis conditions (10 bar of N 2 at 460 °C for 1.5 h) were defined to achieve a pitch with 93% mesophase content, labelled PP-AC. After the pyrolysis, the pitch was grounded in a ball mill to obtain a particle size <500 μm. The powder was physically mixed with anhydrous KOH (activating agent) in a 6:1 ratio (wt.%/wt.%) and immediately heat treated under a nitrogen flow (100 ml min −1 ) at 800 °C for 2 h (heating rate 5 °C min −1 ). The resulting material was washed, first with a HCl solution (10 wt.%) and finally with distilled water. The final sample, labelled PP-AC, was dried overnight at 100 °C. To make the hydrate structures, the nanoporous carbon sample was humidified under water-supplying conditions denoted by R w ( R w , which represents the mass of water to dry carbon). The lower R w values (0.6, 1.1 and 1.8) were achieved by placing the dry carbon in a close container with 90% relative humidity (relative humidity was obtained using a water solution of 34 wt.% glycerine). The larger R w values (2.9 and 4.1) were reached by adding drops of water directly to the sample. Sample characterization Textural properties of the synthesized samples were evaluated by gas physisorption of nitrogen at −196 °C. Gas adsorption measurements were performed in a homemade fully automated manometric equipment designed and constructed by the Advanced Materials Group (LMA), now commercialized as N 2 GSorb-6 (Gas to Materials Technologies; www.g2mtech.com ). The sample was previously degassed for 4 h at 250 °C under vacuum (10 −3 Pa). Nitrogen adsorption data were used to determine the following: (i) the total pore volume ( V t ) at a relative pressure of 0.95, (ii) the BET-specific surface area ( S BET ) and (iii) the micropore volume ( V N2 ) by application of Dubinin–Radushkevich equation. The difference between V t and V N2 is considered to be the mesopores volume ( V meso ). The pore size distribution was evaluated by applying the quenched solid density functional theory method (slit-shape pore-equilibrium model) to the nitrogen adsorption data. The macroporosity of the samples was tested by Hg porosimetry measurements using an Autopore IV 9500 v1.07 porosimeter (Micromeritics, USA). Water adsorption isotherms were measured at 2 °C in a homemade fully automated equipment designed and constructed by the LMA group, now commercialized as Vstar by Quantachrome Instruments. High-pressure analyses were performed in a homemade fully automated manometric equipment designed and constructed by the LMA group, now commercialized as iSorbHP by Quantachrome Instruments. CH 4 adsorption capacity was measured at 2 °C and up to 10 MPa. Dry samples were outgassed at 250 °C for 4 h, while the wet samples were frozen at −20 °C before the outgassing treatment to avoid water loss. Transmission electron microscopyanalyses were performed on a JEOL JEM-2100 F microscope. INS experiment INS experiments were performed at TOSCA spectrometer at the pulse neutron source of ISIS at Rutherford Appleton Laboratory in United Kingdom. Before the experiment, 2 g of dry PP-AC were humidified with deuterated water up to a carbon/water ratio, R w =4.1. The wet sample ( ca. 10.2 g) was wrapped in an Al-foil and loaded into the high-pressure reactor supplied by ISIS. The reactor and the stainless steel pipelines were surrounded by a resistance wire that allows a good temperature control. The sample holder was placed in a 2 m reactor where neutron beam converges. Before the analysis, the sample was kept in contact with methane gas at 2 °C for 1 h. Shortly after that the reactor was properly cooled down to −268 °C with a cryostat. Finally, the reactor was impacted by the neutron beam (150 μA) at −268, −253 and −233 °C. Synchrotron XRPD experiments XRPD experiments were collected at the high-pressure end station of the MSPD beamline at synchrotron ALBA in Spain, using a Rayonix SX165CCD camera and a wavelength of 0.4243 Å. The experiments were performed on an ad hoc capillary reaction cell (fused silica capillary, inner diameter 247 μm, outer diameter 662 μm). Before the experiment, the D 2 O-containing carbon sample was placed inside of the capillary connected to the methane gas cylinder (purity 3.5) via a pressure regulator. An Oxford Cryostream 700 was used to control the temperature of the sample. In situ XRPD measurements were performed at 0, 3 and 5 MPa of methane and two different temperatures, −3 and 2 °C. How to cite this article: Casco, M. E. et al . Methane hydrate formation in confined nanospace can surpass nature. Nat. Commun. 6:6432 doi: 10.1038/ncomms7432 (2015).